Predictive codes of familiarity and context during the perceptual learning of facial identities Face recognition is a key component of successful social behaviour. However, the computational processes that underpin perceptual learning and recognition as faces transition from unfamiliar to familiar are poorly understood. In predictive coding, learning occurs through prediction errors that update stimulus familiarity, but recognition is a function of both stimulus and contextual familiarity. Here we show that behavioural responses on a two-option face recognition task can be predicted by the level of contextual and facial familiarity in a computational model derived from predictive-coding principles. Using fMRI, we show that activity in the superior temporal sulcus varies with the contextual familiarity in the model, whereas activity in the fusiform face area covaries with the prediction error parameter that updated facial familiarity. Our results characterize the key computations underpinning the perceptual learning of faces, highlighting that the functional properties of face-processing areas conform to the principles of predictive coding. The ability to recognize the identity of individuals from their facial appearance is a key component of social interactions. Prerequisite to such abilities is that familiarity increases with a face each time it is perceived, regardless of the viewpoint from which it is being observed [1] , [2] , [3] . Recognition therefore requires continuous and simultaneous updating of the familiarity of a face, and recognition of whether the face has been previously perceived or not based on its familiarity. In dynamic environments facial identities and the viewpoints from which they are observed are perceived in an intermixed manner within context. That is, facial identities are viewed from multiple different angles and are presented in social situations in which they are more likely to be familiar or, conversely, unfamiliar [4] . Yet, there has been little empirical investigation of how view-independent familiarity or contextual effects modulate face recognition. Similarly, there has been no investigation into the neural plasticity that underpins the acquisition of familiarity with faces. We developed a model that made predictions about the computational mechanisms that underpin familiarity acquisition and the evolution of view-invariant representations of faces. This model made predictions about how each presentation of a face increases the likelihood that the same face will be recognized and how such effects will be modulated by context. Predictive coding (PC) accounts of perception suggest that recognition is a function of both contextual information and the learning of stimulus properties. Recent evidence supports the notion that information processing in the visual system can be accounted for by PC mechanisms [5] , [6] , [7] , [8] . In PC information is processed in hierarchically organized sensory systems, with the overarching functional property of the brain being the explanation of incoming sensory information with probabilistically the most parsimonious or efficient model [9] , [10] . Predictive contextual information acts as a top-down influence, with each node within the hierarchy processing expectations about what sensory input there is likely to be. When sensory input is discrepant from predicted input (that is, it is surprising), prediction errors drive learning and pass this information up the hierarchy [8] , [11] . In this framework there are two features that are relevant for the processes of perceptual learning that drive familiarity acquisition. First, context-dependent expectations about likely sensory input will be processed prior to a stimulus and modulate the processing of that stimulus. For face familiarity acquisition, that equates to a prediction about how familiar the upcoming stimulus will be. The importance that is placed on this contextual information in PC sets it apart from other models of learning and attention in which recognition is tied directly to the particular characteristics of the stimulus [12] , [13] . Second, perceptual learning must occur when facial identities are repeatedly presented, in order that future presentations of the face are less surprising. Familiarity with facial identities should therefore be acquired independently of context and viewpoint, in order that the presentation of the same face from any angle is less surprising in the future. However, no study has examined whether faces become familiar and recognized in a manner that conforms to the assumptions of a PC account. Here we developed a computational model of face recognition around the assumptions of PC [11] , [14] , [15] , to examine how contextual and viewpoint independent information influence face recognition and its neural underpinnings. Previous neuroimaging studies have identified a cortical network that is specialised for processing faces, which responds more to faces than any other category of stimulus [4] , [16] , [17] . Within this core face perception network, the fusiform gyrus (specifically the fusiform face area or FFA) and a portion of the superior temporal sulcus (STS) are purportedly important for the process of recognizing the identity of faces [18] . Neuroimaging studies have highlighted how each of these areas show differential responses for correct versus incorrect face recognition and for familiar compared with unfamiliar faces processing [19] , [20] , [21] . In addition, these areas have been shown to respond, to a certain degree, to faces regardless of the viewpoint from which they are being perceived [22] , [23] . This evidence highlights these regions as candidate areas for updating the familiarity of faces and processing contextual information about how familiar a face is likely to be. There were three main aims of this study: first, to investigate how view-independent and contextual effects impact upon face recognition; second, to investigate how activity in the FFA and the STS changes during the acquisition of familiarity with a face independently of viewpoint and third, to test whether the evolution of activity in the these areas can be accounted for by a PC-based computational model. Participants were presented with one face on each trial from a set of 24 unfamiliar facial identities while undergoing fMRI. On each trial, participants were presented with one of the facial identities, from one of three different viewpoints. They were required to indicate whether they had seen the ‘person’ before in the experiment or not. Fifteen of the facial identities were presented from each viewpoint four times. The remaining nine faces were presented once from only one viewpoint. Participants were therefore able to monitor the trial-by-trial view-independent familiarity of the face that was being perceived, but they were also able to process information about how familiar the faces had been on previous trials, that is, the contextual familiarity. To analyse choice behaviour we used a computational model in which the familiarity of each facial stimulus was a function of the view-independent familiarity multiplied by the contextual familiarity. Both of these factors were updated each time a face was presented by ‘prediction error’ parameters that conformed to the assumptions of PC. We fitted the parameters output by the model to neural activity at the time that the faces were presented. As was hypothesised the computational model predicted recognition choices on the task suggesting that face recognition is dependent on both facial familiarity and contextual information. In addition, activity in the FFA and STS covaried with the contextual familiarity and the updating of facial familiarity, respectively. These findings highlight that the mechanisms outlined in PC may be fruitful explicators of the computational and neural processes that underpin face recognition. Behavioural results Participants were presented with one facial identity from a set of 24 on each trial, 15 of which were repeated 12 times across the experiment, four times from each of three different viewpoints. They were required to indicate whether they recognized the identity of the face or not ( Fig. 1 ). Participants showed a clear learning effect, with number of ‘yes’ responses increasing the more times that a facial identity had been presented ( Fig. 2 ). A one-sample t -test showed a significantly higher number of ‘yes’ responses for the last three presentations of each face, compared with the first three presentations of the faces ( t (14)=14.661, P <0.0001). Such effects could not be accounted for by subjects responding ‘yes’ more as the experiment progressed, as novel faces were presented throughout (see Methods). In addition, the familiarity of faces varied considerably over the experiment ( Fig. 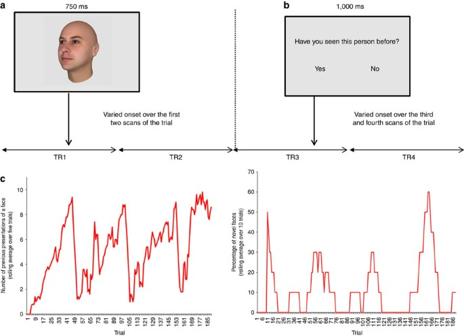Figure 1: Trial Structure and trial order. (a) Each trial began with a 750 ms face stimulus. This cue consisted of a single, coloured FaceGen stimulus provided by the Social Cognition and Social Neuroscience Laboratory, Princeton51. The presentation of the face stimuli were jittered over the first two TRs (TR=3s) of each trial. The faces could be presented front on, 30° from the left (as above) or 30° from the right. The face stimuli were followed by a trigger cue (1,000 ms), which was jittered over the third and fourth TRs of each trial, at which point participants indicated their response on a keypad. This design allowed us to sample activity at the time of the face stimuli independently from activity at the time of the trigger cue. The positions of the ‘yes’ and ‘no’ in the trigger cue were randomly assigned to the left and right of the screen. Participants indicated the left response with their first finger and the right response with their second finger. (b) Variability in the contextual familiarity was introduced by varying the average number of previous presentations of faces over a rolling average of five trials. When the rolling average of the number of times previous faces had been seen was high, the contextual familiarity could be considered as high andvice versafor low contextual familiarity. (c) Varying rate of novel faces over trials displayed as the rolling average of novel faces, regardless of viewpoint over trials. The first ten trials are displayed as zero, to reflect the absence of a rolling average over 10 trials for these first stimuli. 1b,c ) Figure 1: Trial Structure and trial order. ( a ) Each trial began with a 750 ms face stimulus. This cue consisted of a single, coloured FaceGen stimulus provided by the Social Cognition and Social Neuroscience Laboratory, Princeton [51] . The presentation of the face stimuli were jittered over the first two TRs (TR=3s) of each trial. The faces could be presented front on, 30° from the left (as above) or 30° from the right. The face stimuli were followed by a trigger cue (1,000 ms), which was jittered over the third and fourth TRs of each trial, at which point participants indicated their response on a keypad. This design allowed us to sample activity at the time of the face stimuli independently from activity at the time of the trigger cue. The positions of the ‘yes’ and ‘no’ in the trigger cue were randomly assigned to the left and right of the screen. Participants indicated the left response with their first finger and the right response with their second finger. ( b ) Variability in the contextual familiarity was introduced by varying the average number of previous presentations of faces over a rolling average of five trials. When the rolling average of the number of times previous faces had been seen was high, the contextual familiarity could be considered as high and vice versa for low contextual familiarity. ( c ) Varying rate of novel faces over trials displayed as the rolling average of novel faces, regardless of viewpoint over trials. The first ten trials are displayed as zero, to reflect the absence of a rolling average over 10 trials for these first stimuli. 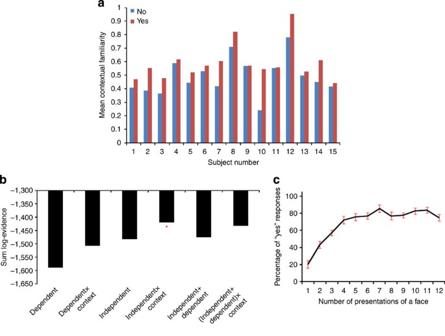Figure 2: Behavioural results showing the winning model and the impact of contextual familiarity on choice. (a) The mean contextual familiarity (yaxis) scaled between zero and 1 estimated by the model was higher on trials when subjects (xaxis) chose ‘yes’ (red) compared with when they chose ‘no’ (blue) in all subjects. All subjects show this effect. (b) Log-evidence (yaxis) for the different models (xaxis), the more negative the value, the poorer the fit of the model to the data. The red star indicates the best fitting model. ‘Dependent’ models assumed that learning was specific to a particular stimulus and did not transfer across the different viewpoints of the same facial identity. (c) The mean percentage of ‘yes’ responses for each presentation of the faces, regardless of viewpoint. Error bars depict the standard error of the mean (n=15). Full size image Figure 2: Behavioural results showing the winning model and the impact of contextual familiarity on choice. ( a ) The mean contextual familiarity ( y axis) scaled between zero and 1 estimated by the model was higher on trials when subjects ( x axis) chose ‘yes’ (red) compared with when they chose ‘no’ (blue) in all subjects. All subjects show this effect. ( b ) Log-evidence ( y axis) for the different models ( x axis), the more negative the value, the poorer the fit of the model to the data. The red star indicates the best fitting model. ‘Dependent’ models assumed that learning was specific to a particular stimulus and did not transfer across the different viewpoints of the same facial identity. ( c ) The mean percentage of ‘yes’ responses for each presentation of the faces, regardless of viewpoint. Error bars depict the standard error of the mean ( n =15). Full size image We fitted a computational model to participant choices (see Methods), in which decisions were assumed to be guided by the overarching level of familiarity ( F ) with a stimulus. This overarching familiarity was calculated as a function of the view-independent familiarity ( V ) (that is, the level of familiarity with a facial identity) multiplied by the context-dependent familiarity ( C ). C is the likelihood that a face will be recognized depending on the view-independent familiarity of facial stimuli on the preceding trials (for example, if the last five facial stimuli have had a high level of view-independent familiarity, then the context-dependent familiarity will be high, increasing the likelihood that participants will indicate that they recognize a face). Each of these two factors is updated by delta-learning rules in a manner that conformed to the principles of PC (Methods). That is, view-independent familiarity was updated by calculating the discrepancy between the current view-independent familiarity with a facial identity and the maximum familiarity of a facial identity (we refer to this difference signal as the view-independent update, δ ), multiplied by an idiosyncratic learning rate parameter ( α ). The context-dependent familiarity was updated by a prediction error parameter ( ε ) that was calculated as the discrepancy between the current view-independent familiarity of a stimulus ( V ) and the context-dependent familiarity of faces on preceding trials ( C ), multiplied by an idiosyncratic free parameter. To ensure that this model was a good fit to the behavioural data, we also compared its fit with the data with five other ‘control’ models (see Fig. 2b and Supplementary methods ). t -tests between the winning model in which behaviour was a function of view-independent and context familiarity had a significantly higher negative log-evidence ( Fig. 2 ) than all of the control models ( n =15, P <0.05, FDR) apart from one, in which the overall familiarity with a stimulus was a function of the view-independent familiarity, the view-dependent familiarity (that is, the familiarity of a face from the particular view it is being perceived from) and context-dependent familiarity. However, this control model contained a larger number of free parameters and therefore its explanatory power is artificially boosted due to its greater complexity. Despite this boosted explanatory power, its summed log-evidence across participants was still lower than the experimental model and thus, our experimental model reflected the most parsimonious account of behaviour on the task. To determine whether the experimental model significantly explained the participants’ choices, we correlated the overall familiarity ( F ) for each trial with the choices made by each subject. A Spearman’s rank test revealed highly significant correlation between these two factors ( n =15, R 2 =0.41, P <0.0001). Thus, a model in which facial familiarity is acquired independently of viewpoint and decisions are made based on the ongoing context-dependent familiarity significantly correlates with the behaviour of participants on this face recognition task. To identify whether the two components of our model (the view-independent familiarity ( V ) and the context-dependent familiarity ( C )) predicted choices on the task we performed a logistic regression between the values of these parameters and choices on every trial. The two variables were entered as predictors in a stepwise manner such that V was entered after C to identify whether V predicted choices and C was entered after V to identify whether C predicted choices. As such, only the variance unique to each was examined when examining their predictive power. To test whether there was a significant effect at the group level, we took the betas output by the single-subject regressions and performed a t- test between these betas and zero. We found that both V ( n =15, t (14)=6.669, P <0.001) and C ( n =15, t (14)=3.417, P <0.004) showed a significant effect. Thus, both components of our model independently predict choices on the task. That is, both learning the familiarity of a face and also the contextual influence of the familiarity of other recently perceived faces influences the likelihood of recognition. An important feature of our hypotheses is that we argue that previously perceived stimuli, even when they are different facial identities, influence choice behaviour. Our model therefore predicts that responses on trials should be consistent with responses on previous trials and also that choice behaviour is influenced by previous stimuli, even when a stimulus being perceived violates the context instantiated by preceding trials. To test the first of these tenets and highlight the effects of context on choice behaviour, we analysed the consistency between responses on a given trial ( n ) and responses on previous trials ( n −1, n −2, n −3 and n −10). We calculated the ratio of ‘yes’ or ‘no’ responses that were consistent with the responses on a previous trial and baseline-corrected this measure by the percentage of ‘yes’ trials across the whole experiment or the percentage ‘no’ trials in the experiment depending on what the response was on trial n. This enabled us to calculate the percentage of trials that were consistent or inconsistent with responses on previous trials without bias. A one-sample t- test revealed that responses on n −1 trials were significantly more consistent with responses on trial n (mean=8.2%, s.e.m.=±3.43) than predicted by chance ( n =15, t (14)=2.415, P <0.05). Responses on n−1 trials were significantly more consistent with responses on trial n than responses on trial n −3 ( n =15, t (14)=2.272, P <0.05FDR) or n −10 trials ( n =15, t (14)=3.664, P <0.05 FDR). Responses on n −2 trials were also significantly more consistent than predicted by chance. These results support the notion that responses on trials were consistent with responses on the immediately preceding trials more than any other, supporting our claim that context influences recognition. Our model predicts that responses to stimuli that are of equal view-independent familiarity should be different when the view-independent familiarity is congruent or incongruent with the contextual familiarity. To examine this effect, we analysed the number of ‘yes’ responses on ‘catch trials’ where the levels of view-independent and contextual familiarity were incongruent, with the responses on trials where these two factors were congruent. To define the catch and non-catch trials, we calculated the running average (over five trials) of the number of times a face had been seen previously during the experiment. This is a corollary of the level of contextual familiarity over trials. We then selected the trials where the number of times the face had been presented previously during the experiment was (A) more than four times greater than the rolling average and (B) more than four times less than the rolling average. This gave us the catch trials where the model would predict a bias towards responding (A) ‘yes’ or (B) ‘no’ as a result of contextual familiarity. There were 10 trials that fell into each of these categories. To compare these with comparable trials where the level of familiarity of stimuli and the contextual familiarity were congruent, we picked the trials where the number of times the face had been presented was within two of the rolling average in high and low contextual familiarity conditions. This created four trial-types: congruent high contextual familiarity (where over the previous five trials, the average number of times the faces had been presented previously during the task was high (mean=10.3) and the facial identity on on trial n had been presented on average 10.3 times during the experiment); incongruent low contextual familiarity (where the identity presented on trial n had been presented on average 10.2 times during the experiment, but over the previous five trials, the average number of times the faces had been presented previously during the task was low (mean=4.6)); congruent low contextual familiarity (where the identity presented on trial n had been presented on average only 1.5 times previously during the experiment and over the previous five trials, the average number of times the faces had been presented previously during the task was also low (mean=1.98)); and incongruent high contextual familiarity (where the facial identity on trial n had been presented on average 1.5 times during the experiment, but over the previous five trials, the average number of times the faces had been presented previously during the task was higher (mean=6.2)). Our model would predict that contextual information would bias ‘yes’ responses on the task when the contextual familiarity was higher than the familiarity of the stimulus and bias ‘no’ responses when the contextual familiarity was lower than the familiarity of the stimulus. In line with the first of these predictions, a t -test revealed significantly more ‘yes’ responses on the congruent high contextual familiarity ( M =83%) trials as compared with the incongruent low contextual familiarity ( M =67%) condition ( n =15, t (14)=3.055, P <0.005 FDR). As such, when previously seen faces had been less familiar than a face being perceived, the subjects were less likely to recognize the stimulus than when an equally familiar stimulus was seen in the context of high familiarity. A t- test did not show any significant differences between the congruent low contextual familiarity and the incongruent high contextual familiarity ( n =15, t (14)=0.636 P >0.05 FDR). However, broadly speaking, the first result provides further behavioural evidence in support of the effects of context and validation of our model. fMRI results We examined activity time-locked to the face stimuli and performed a parametric analysis. We took a region of interest (ROI) approach and examined activity in three regions within the core face perception network that were identified by a localizer ( Supplementary Fig. S1 ). This included the right STS and bilateral FFA. The aim of the study was to identify whether activity in these regions covaried with parameters from the computational model. We tested whether the activity in these regions could be explained by any of the following parameters: first, the overall familiarity ( F , view-independent familiarity ( V ) × context familiarity ( C )); second, the view-independent familiarity ( V ); third, the view-independent update ( δ , the discrepancy between view-independent familiarity for that identity and the maximum familiarity); fourth, the context-dependent familiarity ( C ) and fifth, the context-dependent prediction error ( ε , discrepancy between the predicted and actual familiarity of a face). In line with our hypotheses, t -tests revealed that activity in the FFA and in the STS covaried significantly with only one of the parameters from the computational model. Activity in both the right ( n =15, t (14)=4.405, P <0.0005) and left ( n =15, t (14)=9.661, P <0.0001) FFA was found to vary parametrically with the view-independent update parameter ( δ ) in the model ( Fig. 3 ). t -tests between the beta coefficients of this parameter and each of the other parameters from the model showed a significant difference between each parameter and the view-independent update parameter in both the right and left FFA ( n =15, P <0.05 FDR). A random-effects (RFX) group analysis supported this finding, identifying activity bilaterally within the FFA that covaried with the independent-update parameter from the model ( Fig. 3 ). 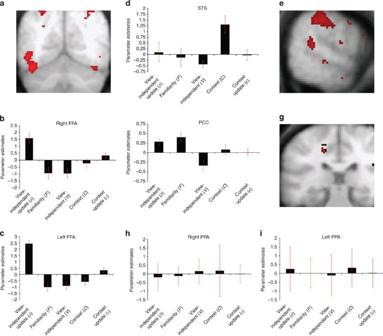Figure 3: fMRI results showing activity correlating with parameters from the model. Activity shown in brain areas targeted for ROI analysis. Clusters shown are taken fromt-tests (n=15) on the complimentary random-effects analysis. Activity shown in (a) the right (46, −56, −26,Z=2.5,P<0.05 svc) and left FFA (42, −66, −16,Z=2.8,P<0.05 svc) covarying with the parameter that updated the familiarity of the face. Activity shown in the STS (e) covarying with the contextual familiarity from previous trials (66, −24, −4, Z=3.24,P<0.05 svc). Activity shown in the PCC (g) covarying with the overall level of familiarity that drove recognition judgements. Plots of the contrast estimates for each of the five parameters from the model for the (b) right FFA (c) the left FFA (d) the STS and the (f) PCC from the ROI analysis. Additional plots from the right (h) and left (i) PPA showing that activity in this area did not covary with any of the parameters from the model. Error bars depict the s.e.m. Figure 3: fMRI results showing activity correlating with parameters from the model. Activity shown in brain areas targeted for ROI analysis. Clusters shown are taken from t -tests ( n =15) on the complimentary random-effects analysis. Activity shown in ( a ) the right (46, −56, −26, Z =2.5, P <0.05 svc) and left FFA (42, −66, −16, Z =2.8, P <0.05 svc) covarying with the parameter that updated the familiarity of the face. Activity shown in the STS ( e ) covarying with the contextual familiarity from previous trials (66, −24, −4, Z=3.24, P <0.05 svc). Activity shown in the PCC ( g ) covarying with the overall level of familiarity that drove recognition judgements. Plots of the contrast estimates for each of the five parameters from the model for the ( b ) right FFA ( c ) the left FFA ( d ) the STS and the ( f ) PCC from the ROI analysis. Additional plots from the right ( h ) and left ( i ) PPA showing that activity in this area did not covary with any of the parameters from the model. Error bars depict the s.e.m. Full size image t- tests revealed activity in the right STS that varied parametrically with the context-dependent familiarity ( C ) parameter ( n =15, t (14)=3.447, P =0.002). t -tests between the beta coefficients of this parameter and each of the other parameters from the model showed a significant difference between each parameter and the context-dependent parameter in the right STS ( n =15, P <0.05 FDR). The RFX analysis also identified a portion of STS in which activity covaried statistically with the independent update parameter ( P <0.05 svc). Importantly, we found no effects of any of our variables in the parahippocampal place area (PPA), an area that responds to objects but not faces, suggesting that our effects were specific to faces in this task ( Fig. 3 ). In addition to the ROI analysis, we performed a RFX analysis that examined activity which covaried with any one of the parameters within the model, beyond the FFA and STS. t -tests revealed activity in the posterior cingulate sulcus (PCC), (BA23c′; MNI coordinates: −18, −30, 40; Z =3.40, P <0.05 svc) that varied with the overall level of familiarity. In summary, we have shown that activity in the FFA correlates with the amount that the familiarity of a face is updated every time it is perceived, while activity in the STS signals the contextual familiarity of recently perceived faces and the PCC signals the overarching familiarity of a stimulus. Becoming familiar with the visual properties of another’s facial features and recognizing their identity regardless of the viewpoint from which they are observed is a key feature of human face recognition. Here we used a computational model that was built around the principles of PC [11] , which allowed us to examine behaviourally whether both view-independent and contextual familiarity influence face recognition. We tested whether the activity in the STS and the FFA at the time that a face is perceived covaried with parameters from the computational model. In line with our predictions, the level of familiarity calculated by the model significantly predicted participants’ choices and also fit the behavioural data better than control models that were based around alternative assumptions. The fMRI results revealed that activity in both the FFA and the STS both covaried exclusively with one of the parameters from the model. The STS covaried with the contextual familiarity of faces on preceding trials, while FFA activity covaried with the parameter that updated the familiarity of each facial identity. These results highlight how face recognition is dependent both upon the view-invariant familiarity of a facial identity and also the context within which the face is perceived. Our results are therefore consistent with the view that faces become familiar and recognized by processing in the FFA and the STS that conforms to the principles of PC. There is considerable evidence that the FFA is activated during the recognition of facial identities [24] . Lesions to this region can cause prosopagnosia [25] , the inability to recognize the identity of familiar individuals, while leaving the ability to detect the presence of a face intact. Numerous studies that have employed fMRI adaptation paradigms have demonstrated the sensitivity of the FFA to differences in face identity [21] , [26] , [27] , [28] , [29] , [30] . In such paradigms the FFA shows a decreased response when one face stimulus is presented twice in rapid succession, when compared with the response when two novel stimuli are presented in the same manner. This adaptation effect is present even when the face is shifted in the field of view, changed in size or spatial scale. This suggests that the FFA is engaged when processing the identity of a face and not by the processing of lower level visual properties. In this study, we did not use a repetition suppression design, but our results support the notion that the FFA processes facial identities. In addition, our results support the findings of neurophysiology studies that have found a region of the inferior temporal cortex, which is homologous to the FFA, that contains neurons in which the spike frequency declines in a non-linear manner over repeated presentations of the same face [31] . Our model would predict such a non-linear decline in activity in the FFA over repeated presentations of the same face. Furthermore, we have shown that this signal relates to the updating of the familiarity of a face and thus the likelihood that the face will be recognised in the future. Despite the evidence from repetition suppression studies indicating that the FFA is sensitive to information about the identity of a face, it has previously been unclear what functional property of the FFA drives such repetition suppression effects [24] . Our results offer a novel interpretation of adaptation in the FFA. In our model, the view-independent update signal declines with each presentation of a stimulus. Each time a face is presented it has become more familiar and thus less updating needs to be performed for the face to be recognized in the future. Accordingly, we predicted and have shown in this study that the signal in the FFA should decline each time the same face is presented. Thus, in a repetition suppression paradigm, when two stimuli are identical our model predicts a large updating signal when the first stimulus is presented and a smaller updating signal when the second, identical face is presented. However, when the second stimulus is novel and distinct from the first face stimulus, the updating signal will be high for both faces. Thus, our model predicts that a greater BOLD signal would be evoked by two different, unfamiliar facial identities than two presentations of the same identity, as is found in the FFA in repetition suppression studies [29] . The results of our study therefore suggest that facial identity adaptation effects in the FFA may in fact be a result of differences in the amount of familiarity updating that occurs when stimuli are repeated compared with when stimuli are novel. It is notable that previous studies have found that activity in the FFA is sometimes dependent upon the viewpoint from which the face was first perceived [32] , [33] . In contrast, our study suggests that FFA activity is view-independent. How can these two findings be reconciled? We argue faces are rarely seen from one static viewpoint. Therefore, while the FFA may contain neurons that respond in a view-dependent manner, in dynamic environments, these responses will be combined at the population level into a response that is view-independent. Thus, sensitivity to both view-dependent and view-independent information in the FFA is consistent with our claims that this region is engaged when updating the familiarity of a face. We observed that activity in the FFA correlates with the amount that the familiarity of a face is updated. This would suggest that activity in the FFA will be higher for faces that are unfamiliar than familiar, which largely contradicts previous accounts that argued that FFA activity should be greater for familiar compared with unfamiliar faces, if it is involved in identity recognition [34] . A neuroimaging study using personally unfamiliar facial stimuli, which then became familiar during a learning session, supported the notion that FFA processes a familiarity updating signal, with greater activity evoked by unfamiliar than familiar faces in the testing session [19] . The only previous study that investigated changes in the BOLD response over repeated presentations of faces also reported a decrease in activity in the FFA over time for the faces that were repeated across sessions [35] . However, in that study activity was measured across blocks of stimuli and across sessions and not specifically at the time of each face stimulus, as was the case in our study. In contrast, studies using personally familiar faces and faces of celebrities, report either greater activity for familiar faces or no difference between familiar and unfamiliar faces in the FFA at all [34] , [36] , [37] . We argue that such effects may be result of inherent the difficulties in comparing the visual familiarity of such stimuli. We suggest that the FFA is engaged when the visual properties of the face are updated and not by any form of affective, cognitive or autobiographical familiarity. Such an account would be consistent with the mixed findings in studies of face familiarity processing, where controlling for the visual familiarity of faces is almost impossible. Recent studies also highlight how the FFA processes information in a manner that conforms to the principles of PC [5] , [6] , [7] , [38] . In these studies the FFA was shown to process predictions and prediction errors for the presence of a novel face stimulus, when face and house stimuli were intermixed. Thus, in those studies the activity in the FFA was driven by the detection of faces as opposed to recognition of faces. In our study, where all stimuli were faces, the processing was specific to face recognition rather than detection. This is consistent with the established notion of the FFA having a dual-role in both recogtion and detection [24] . Thus, the conjunction of our results and previous studies investigating PC mechanisms reveal that both face detection and recognition may be accounted for by PC processes operating within the FFA. In addition, our results extend upon previous studies investigating PC by providing the first empirical support for the notion that perceptual learning processes in regions, which are specialized for processing particular categories of stimuli, conform to similar computational principles as those underpinning attention and stimulus detection [8] , [39] , [40] . Perhaps the most novel of our findings is that the STS processes contextual information about stimulus familiarity [24] . The STS contains patches of cells that are face-selective in monkeys [3] , [41] . In human neuroimaging repetition suppression studies the posterior portion of the STS is known to be sensitive to gaze direction and emotional expressions [42] , but also shows sensitivity to facial identities [21] , [28] . If the STS processes such a variety of different types of information about faces, what is its role is face perception? Our results suggest that an important function of the STS may be to process predictive information about task-relevant features of faces. In a PC framework, these predictions are probabilistic and are therefore updated by every face stimulus. There is evidence to support the notion that STS flexibly processes contextual information about faces, with several studies showing that information about gaze direction and emotional expressions are only processed in certain circumstances [43] , [44] . Importantly, the STS has been found to show greater activation when contextual expectations about others’ based on their gaze direction or facial expression are violated, in a manner that is akin to prediction error signals in PC [45] , [46] . We therefore argue that an important functional property of face-selective portions of the STS is to process probabilistic task-relevant information about faces in a manner that conforms to the principles of PC. Activity in the PCC covaried with the familiarity of each stimulus as a function of both the view-independent familiarity and the contextual familiarity. This suggests that information about different forms of familiarity converges in the PCC, resulting in activity that is graded with the likelihood that a participant will decide that a face is recognized. Recent reviews of PCC function suggest that its overarching functional property is to signal the salience of information that guides decisions across a broad range of different domains, including face perception [47] . Single-unit recording studies also support this notion by identifying neurons in which the firing properties are graded with the likelihood of a change in choice behaviour [48] , [49] . The same portion of the PCC also contains neurons that respond to the salience of face stimuli [50] . The PCC has also been found to respond more to familiar faces than unfamiliar faces in neuroimaging studies [19] , [35] . These results are therefore consistent with the view that PCC activity is graded with the trial-by-trial familiarity of a stimulus when the task is to decide whether the face has been seen before or not. In conclusion, the results are consistent with the view that familiarity can be acquired with faces regardless of the viewpoint from which they are perceived, but the decision of whether a face will be recognized is also dependent on how familiar recently perceived faces have been. The study highlights that an important functional property of the FFA is to update how familiar a facial identity is. In contrast, the STS processes task-relevant, contextual information about the recent history of the familiarity of faces. These results highlight how the important process of becoming familiar with a face and recognizing its identity may be underpinned by the computations predicted by PC. Participants Participants were 16 (a standard sample size for fMRI research) healthy right-handed participants (aged between 18 and 30; 10 female), screened for neurological and psychological conditions. One (male) subject failed to show a learning effect and become familiar with the facial identities during the experiment. This participant was excluded from the analyses. Subjects were paid £10 for their participation. Subjects gave written informed consent and the study was approved by the Royal Holloway University of London Psychology Department Ethics Committee and the study conformed to regulations set out in the CUBIC MRI Rules of Operations ( http://www.pc.rhul.ac.uk/sites/cubic/ ). Participants took part in an fMRI study that investigated how familiarity is acquired with the visual features of facial identities. Participants were presented with trials ( Fig. 1 ) during which they saw a single Facegen computer-generated facial stimulus (see Supplementary methods for more details) that was presented at one of three different viewpoints [51] . The faces could either be presented front on or at a 30° angle from the left or the right. The participants’ task was to decide whether they had seen that facial identity, regardless of the viewpoint at which it was being shown from or had previously been shown from during the experiment. There were 24 facial identities which the participants were completely unfamiliar with before the experiment. Nine of these identities were presented only once from one viewpoint. Fifteen facial identities were presented 12 times during the experiment, with four repetitions of each identity from each viewpoint. Participants were therefore required to try and recognize faces from novel viewpoints, even if they had not seen that face from the viewpoint before. The order of presentation of the face stimuli was partially pseudorandomized. The order with which each identity was presented from the different viewpoints was randomized, such that the different facial identities were not presented in the same order of viewpoints. However, important elements of the stimulus order were controlled in order to examine, in line with one of the aims of the experiment, the contextual effect of the familiarity of previously perceived faces. To that end, it was important to vary the level of familiarity of faces throughout the experiment. Periodic changes in familiarity were introduced by breaking the trials up into five blocks and controlling the stimulus order in the latter four blocks. Another control on the order of presentations was that novel facial identities were introduced throughout the experiment, such that participants were not able to perform the task more accurately during the experiment by increasing the number of ‘yes’ responses ( Fig. 1 ). Computational modelling To analyse the behavioural responses of participants we used a computational modelling approach. Our aim was to examine whether the behaviour of participants could be accounted for mathematically by a model of facial familiarity acquisition that is underpinned by the assumptions of predictive coding. We created one experimental model that tested specific predictions about the processing of facial familiarity. In addition we developed five control models that tested alternative possible explanations of participants’ responses on the task. This approach allowed us to test whether the behaviour of participants on the task could be accounted for by our experimental model and not by other alternative explanations of how facial familiarity might be acquired. Previous behavioural studies have highlighted how facial familiarity can be acquired partially independently of the view from which the face is first viewed at [52] , [53] . That is, faces can be recognized from one viewpoint, even if they have previously only been viewed from a different viewpoint. As such, familiarity can be acquired with a facial identity and transferred to another viewpoint, to reflect an overarching level of familiarity with a face. We therefore assumed that behaviour on our task would be a function of familiarity that was acquired regardless of the viewpoint from which faces were perceived from. However, predictive coding accounts also highlight the importance of top-down context-dependent expectations about likely sensory input as modulators of behavioural responses [9] . We therefore also assumed that facial recognition will be dependent on the moderating effects of contextual information. We created a model in which the familiarity of a facial stimulus was a function of (i) the view-independent familiarity with the facial identity and (ii) the familiarity of previously viewed faces, that is, how familiar the faces were on previous trials. Thus, our experimental model assumed that each choice of whether a face is recognized or not will be dependent upon the familiarity of that facial identity moderated by how familiar the recent history of perceived faces. Predictive coding accounts make predictions about how information will be processed in the cortex. One suggestion is that information will be processed in terms of predictions and violations of expectations (prediction errors). For perceptual learning and stimulus recognition to occur, predictive information must reflect the familiarity with a stimulus, and prediction errors the discrepancy between how familiar the stimulus was before it is perceived and how familiar the stimulus will be if it is perceived in the future [8] , [11] . We therefore created a model in which the view-independent familiarity and the contextual familiarity were updated by prediction error signals. In our experimental model, therefore, the overarching familiarity ( F ) of a stimulus is a function of the view-independent familiarity ( V ) multiplied by the contextual familiarity ( C ). On each trial ( t ), the level of familiarity ( F ), and therefore the likelihood of responding that the face is recognized, is a function of the view-independent familiarity of the facial identity (i) being perceived, multiplied by the contextual familiarity. The view-independent familiarity was updated for a facial identity on each trial where that facial identity was perceived. As such, on future trials where the same face was perceived, the familiarity with that face has been updated and is now more likely to be recognized. The view-independent familiarity was assumed to be updated by a simple delta-learning rule: where: where V is the view-independent familiarity of an identity ( i ). n is the number of presentations of each identity from any viewpoint. δ is the updating parameter of the view-independent familiarity. In (3) it is calculated as the difference between the maximum familiarity of any facial identity ( λ ) and the view-independent familiarity of the n th presentation of that identity. It equates to a prediction error signal as found in predictive coding models, where the discrepancy is calculated between the probability of the occurrence of a sensory event and the actual sensory event. The prediction error therefore updates predictions about the likelihood of a sensory event occurring following an actual sensory event. However, in our model, we calculate the discrepancy between the current familiarity of an individual’s face and the maximum familiarity of a facial identity. This discrepancy signal is then added to the current familiarity of that identity, such that that the familiarity of a facial identity is increased, increasing the probability that the face will be recognized the next time it is perceived. To account for individual differences in the rate at which individuals learn to recognize faces, we multiplied the independent update parameter by α , an idiosyncratic free parameter which was scaled between zero and 1. This scaled the rate at which familiarity was acquired with the facial identities. To reflect the fact that participants made false positive responses, that is, they responded ‘yes’ to facial identities that had not previously been seen, the initial value of V for all of the identities was set idiosyncratically for each participant. We defined the initial value of V as the percentage of false-positive responses on the 24 stimuli that were the first presentations of each face, multiplied by λ , the maximum familiarity parameter. The initial value of V therefore reflected the baseline level of familiarity as a function of how familiar faces could become for that participant during the experiment. It is important to note that the asymptotic value of familiarity is used to calculate the view-independent familiarity updating signal. We therefore make the assumption that the subject is calculating the difference between the maximum familiarity of a face and its actual familiarity, before the maximum level of familiarity with that face is known. We suggest that this maximum familiarity is developed ontogenetically and reflects a tuning property of neurons involved in the perceptual learning of facial identities. As such, we suggest that this asymptotic value is akin to the values calculated in the Rescorla–Wagner model in reinforcement learning [13] , [54] , [55] , [56] , [57] and the Pearce–Hall [12] algorithm in attention-based error learning, which have been shown to be effective models of other types of learning. To model contextual effects we multiplied the trial-by-trial view-independent familiarity by a context-dependent parameter ( C ). This contextual parameter was also updated by a delta-learning rule. However, this delta-learning rule was updated on every trial, regardless of the identity of the face: where: In (4) C is the contextual familiarity on trial (t). This is updated such that the contextual familiarity on the next trial will be a function of the current contextual familiarity added to the ‘prediction error’ ( ε ) multiplied by an idiosyncratic learning rate ( δ ). The prediction error is calculated as the difference between the current contextual familiarity on that trial ( C ) and the view-independent familiarity of the current stimulus. The learning rate parameter therefore dictates how sensitive the participant is to trial-by-trial changes in the familiarity of facial stimuli. The updating signals in this model are akin to the prediction error signals that are an important component for how information is updated in PC. We note that most formulations of PC rely on Bayesian principles [14] , [58] , an approach that we have not employed in this study. There are multiple formulations of PC that use different Bayesian-based approaches to model surprise signals and perceptual learning [11] . Testing each of the alternatives would not be possible within the scope of one study. Thus, we used a model which tested whether behaviour and activity in the brain could be explained by the basic principles that are common to all PC formulations. We were therefore able to test whether the underlying assumptions of PC can account for face-recognition processes. Model estimation To fit the experimental model to the data, the familiarity ( F ) needed to be converted to a probability that would reflect the likelihood that the participant would recognize the facial stimulus and respond ‘yes’. To do this we used a Luce choice rule, which has previously [59] , [60] been used for fitting models to two alternative choice tasks in both economic and psychological tasks, to calculate the probability that the familiarity would lead to a ‘yes’ response: To calculate the probability of a ‘no’ response we calculated The Luce choice rule converts the Familiarity ( F ) on each trial to a probability, such that higher values of F reflect an increased probability of participants recognizing a face. If the participant made a ‘yes’ response, then P was calculated as in (6). If the participant’s response was ‘no’ then P was calculated as the inverse of P yes ( t ). In (6) β is an idiosyncratic free parameter that reflects the stochasticity of the participants choices on the task, and therefore their sensitivity to the value of F (t). The model we used in this experiment contained several free parameters that we estimated separately for each participant. To fit the model to the data we used a maximum likelihood approach. We varied each parameter within a set range to identity the set of parameters that optimally explain the choices of each participant on the task. We varied the view-independent learning rate parameter ( α ) between 0 and 1 in steps of 0.01, the context-dependent learning rate ( δ ) between 0 and 1 in steps of 0.01, the maximum familiarity ( λ ) between 0 and 2 in steps of 0.01 and we varied the stochasticity parameter ( β ) between 0.1 and 20 in steps of 0.1. The output of the Luce choice algorithm is a series of probabilities, based on the values of each of these parameters and the choices made by the participant. To select the parameters that best fitted the choice behaviour, a maximum likelihood approach was used. By using a maximum likelihood algorithm it was possible to maximize the probabilities of the choices made by the subjects and estimate the values of each of the parameters that produced the behaviour. where the likelihood of each set of parameters ( L ) is determined by the log of the probability of the chosen response ( P a ) at trial t, according to the model. If the model perfectly predicts the responses, the probability of every chosen response would equal 1 and L would be 0. As the probabilities become <1 the log-likelihood L assumes negative values. The best fitting parameters were then selected using: This identified the set of parameters for which L was closest to 0, that is, the best fitting parameter set. Where θ is the parameter set and L is the log-likelihood. In addition to this main experimental model we also created five control models. Each of the models assumed that each presentation of a stimulus updates familiarity with stimuli on future trials within a delta-learning framework. However, the factors that drove the familiarity in each of the models were distinct from the experimental model. Two of these models assumed that behavioural responses would not be dependent on contextual effects but only on properties of each perceived stimulus ( Supplementary methods ). Thus, they approximated to error-learning models of attention, such as the Pearce–Hall formulation [12] . Each of the five control models were fitted to the behavioural data using a maximum likelihood approach, in the same manner that the experimental model was fitted. This enabled us to compare the fit of each of the models in terms of the log-evidence using post hoc t -tests ( Supplementary methods ). Region of interest analysis The aim of our analysis was to define regions of interest (ROIs) for the STS and the FFA and analyse whether activity in these regions covaried with the parameters from the experimental model. In order to determine ROIs for each individual participant, we contrasted activity associated with face blocks with that associated with house blocks in the localizer. Results of this contrast were thresholded flexibly (from uncorrected P <0.05 to P <0.00005, cluster-size>10 voxels) in order to identify and isolate in each subject clusters of face-sensitive voxels on the fusiform gyrus, and the STS (see Supplementary Fig. S1 and Supplementary Table S2 ). In addition, we also defined ROIs in the same manner in the PPA. The PPA acted as a control region as its activity should not vary with any of the parameters of our experimental model, if activity in the task is driven by familiarity with the identity of the face. We extracted ROIs in the PPA using the same approach as for the FFA and STS. We obtained bilateral fusiform gyrus and right STS activity in all 15 of the participants. However, we found left STS activity in only 10 participants and an analysis of activity in this region was therefore not possible. In each participant we extracted beta estimates for the parametric modulators in each of the five GLMs in each of the three regions using Marsbar software. We then performed post hoc t -tests in each region between the parametric modulators that had the highest mean beta values across participants and the beta values of each of the other parametric modulators. To correct this analysis for multiple comparisons we employed a Benjamini–Hochberg false discovery rate (FDR) procedure within each region. Random-effects analysis In addition to the hypothesized activity in the FFA and STS, we also performed a group analysis to identify whether additional regions also process information in a manner that conforms to the predictions of the computational model. A random-effects analysis was applied to determine voxels in which activity varied significantly at the group level. SPM{t} images for each of the five parametric modulators from all subjects at the first-level were entered into second-level design matrix. To identity whether activity in any area covaried exclusively with one of the parameters from the model we performed t -contrasts between each of the parameters and each of the others. We only report a region as activated if activity in this region covaried significantly with one of the parameters (see Supplementary Table S1 for a full list of results at a reduced thereshold) and if that parameter explained activity in that region significantly better than all of the other parameters. This approach additionally enabled us to confirm the results in the FFA and STS at the group level. A random-effects analysis was employed on the localizer experiment. To correct for multiple comparisons at the group level for the main experiment, we used a mask of the t -contrast Face>House ( n =15, P <0.001 uncorrected) from the localizer group analysis. This allowed us to correct for multiple comparisons in the random-effects analysis in the main experiment, by the number of voxels that showed a group-level difference between faces and houses in this sample of participants. It also allowed us to restrict our results spatially such that we only identified voxels that showed facial specificity at the group level. How to cite this article: Apps, M.A.J. et al. Predictive codes of familiarity and context during the perceptual learning of facial identities. Nat. Commun. 4:2698 doi: 10.1038/ncomms3698 (2013).